Enhancing the fidelity of neurotransmission by activity-dependent facilitation of presynaptic potassium currents Neurons convey information in bursts of spikes across chemical synapses where the fidelity of information transfer critically depends on synaptic input–output relationship. With a limited number of synaptic vesicles (SVs) in the readily releasable pool (RRP), how nerve terminals sustain transmitter release during intense activity remains poorly understood. Here we report that presynaptic K + currents evoked by spikes facilitate in a Ca 2+ -independent but frequency- and voltage-dependent manner. Experimental evidence and computer simulations demonstrate that this facilitation originates from dynamic transition of intermediate gating states of voltage-gated K + channels (Kvs), and specifically attenuates spike amplitude and inter-spike potential during high-frequency firing. Single or paired recordings from a mammalian central synapse further reveal that facilitation of Kvs constrains presynaptic Ca 2+ influx, thereby efficiently allocating SVs in the RRP to drive postsynaptic spiking at high rates. We conclude that presynaptic Kv facilitation imparts neurons with a powerful control of transmitter release to dynamically support high-fidelity neurotransmission. Classical work by Hodgkin and Huxley [1] ingeniously described single action potentials (APs or spikes) in the squid giant axon with mathematical expressions of intricate time- and voltage-dependent changes in two conductances: Na + and K + conductance. However, overwhelming evidence suggests that central neurons integrate a large number of ion channels to generate single APs and more complex patterns of spikes to encode information [2] , [3] , [4] , [5] , [6] , [7] , [8] , [9] , [10] , [11] . Among these channels, K + channels are the most diverse of all, containing 10 subfamilies with a total number of subunits exceeding 70 (ref. 12 ). Different combinations of subunits from the same and/or different subfamily of K + channels give rise to tremendous heterogeneity in neuronal excitability, spike waveform and firing patterns manifested by distinct populations of neurons in the mammalian brain. Aside from the diversity of native K + channels, functional and structural studies have further extended the simple gating states that Hodgkin and Huxley [1] originally implicated (that is, 0–4 gating particles) to show that each channel gates in much more complicate schemes. Indeed, computational modelling of K + and other ion channels suggest that highly dynamic transition between multiple gating states, including several closed states, open state and in some cases inactivation states, takes place to account for macroscopic behaviour of ion channels that underlies various forms of firing activity typically recoded from soma or dendrites of neurons [3] , [4] , [5] , [8] , [9] , [10] , [11] , [13] . However, very little is known about whether and how the intermediate gating states of voltage-gated channels contribute to the presynaptic excitability and transmitter release in a physiological context. To this end, we investigate the properties of voltage-gated K + channels (Kvs) at the calyx of Held nerve terminal in the mouse brainstem and several other fast-spiking neurons in hippocampus and cerebellum with short bursts of native or pseudo-APs. We find that currents mediated by Kvs facilitate in a frequency-dependent but Ca 2+ -independent fashion. With further experiments and computer simulations using the Markov kinetic modelling of ion channels at the presynaptic calyces [14] , [15] , [16] , we reveal that this facilitation resides in the intermediate closed states of Kvs, independent of any diffusible second messengers, and affects the synaptic input–output relationship. Our observations suggest that the enhancement of Kvs fine-tunes presynaptic spikes, and critically regulates the magnitude and polarity of short-term synaptic plasticity to dynamically promote high-fidelity neurotransmission. Neuronal K + currents facilitate during repetitive activity In the mammalian brain, fast-spiking neurons fire regularly at several 100–1,000 Hz with little adaptation, and have crucial roles in gating input detection, integration and information coding. For example, cerebellar Purkinje cells (PCs) and principal neurons in the auditory brainstem rapidly transmit motor and sensory signals with temporal precision, while inhibitory interneurons in the cortical or subcortical areas project strong inhibition to modulate the local network activity important for a variety of cognitive functions. To directly investigate biophysical basis of the fast-spiking modality, we first isolated and recorded K + currents ( I K ) from several fast-spiking central neurons, including hippocampal dentate gyrus interneurons (DGIs), cerebellar stellate neurons (SNs) and PCs, as well as the calyx of Held synapse in the auditory brainstem, under the condition that Na + and Ca 2+ channels were blocked by extracellular tetrodotoxin (TTX; 0.5–1 μM) and cadmium chloride (CdCl 2 ; 20 μM), respectively. We evoked I K by a pair of identical pseudo-APs at incremental intervals with their waveforms mimicking native spikes at room (22 °C) or near-physiological temperature (35 °C) from these neurons ( Fig. 1 and Supplementary Fig. 1 ). Unexpectedly, we found that I K activated by the second spikes significantly enhanced in all cases. 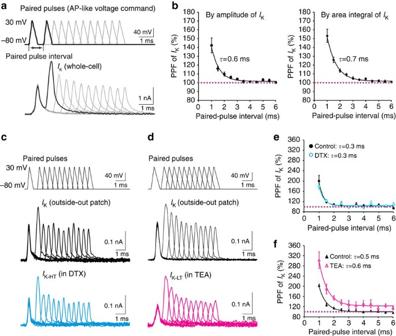Figure 1: Paired-pulse facilitation (PPF) of native K+currents from the central nerve terminal. (a) Potassium currents (IK, bottom panel) obtained from the calyx of Held nerve terminal in the whole-cell mode in response to a pair of action potential (AP)-like voltage command with variable intervals from 1 to 6 ms (AP waveform: −80 to +30 mV, rise time: 0.2 ms, decay time: 0.4 ms, top panel). The inter-pulse interval is illustrated as the time difference between the starting points of two pulses. (b) PPF, defined as the ratio of the amplitude (left) or area integral (right) of the 2ndIKversus that of the 1st responses, declines over increasing time intervals. The decay rates of PPF are fit with a single exponential function and the time constants (n=9) are given in this and following figures. (c,d) Representative traces ofIKrecorded from outside-out patches of the nerve terminal in the absence (black traces, middle panels) or presence of α-dendrotoxin (DTX, blue traces,c) or tetraethylammonium (TEA, magenta traces,d) in response to the paired-pulse paradigms (top panels: amplitude: −80 to +30 mV; half-width: 0.3 ms inc, 0.45 ms ind). (e,f) Summaries of the extent of PPF (quantified by area integral ofIK) with or without DTX (n=6) or TEA (n=7) over inter-pulse intervals. Error bars indicate ±s.e.m. 1st, first; 2nd, second. Figure 1a,b illustrated from the calyx of Held nerve terminal, the amplitude and area integral of I K evoked by the second spike facilitated by 142.4±8.3% (mean±s.e.m.) and 153.3±7.5% relative to that by the first spike at the interval of 1 ms, respectively (AP waveform: −80 to +30 mV, rise time: 0.2 ms, decay time: 0.4 ms). This facilitation decreased as the interval increased and diminished completely within 10 ms. The time-dependent decline in paired-pulse facilitation (PPF) by measuring the amplitude or area integral of I K can be well described by single exponential functions with similar time constants ( τ ) of 0.6 or 0.7 ms ( Fig. 1b ). This phenotype was also evident for I K recorded from hippocampal DGIs, cerebellar SNs and PCs ( Supplementary Fig. 1a–c ). To determine whether PPF of Kvs is restricted to fast-spiking cells, we investigated I K from hippocampal CA1 neurons (CA1s), which are well known for firing at low frequencies. Similar to the fast-spiking neurons, I K in CA1s evoked by a pair of pseudo-APs facilitated and the PPF reduced exponentially over prolonged intervals as well ( Supplementary Fig. 2 ). These observations suggest that Kvs in many types of neurons facilitate, although the extent and decay time course of PPF are different, likely depending on the composition of native K + channels and experimental conditions. Figure 1: Paired-pulse facilitation (PPF) of native K + currents from the central nerve terminal. ( a ) Potassium currents ( I K , bottom panel) obtained from the calyx of Held nerve terminal in the whole-cell mode in response to a pair of action potential (AP)-like voltage command with variable intervals from 1 to 6 ms (AP waveform: −80 to +30 mV, rise time: 0.2 ms, decay time: 0.4 ms, top panel). The inter-pulse interval is illustrated as the time difference between the starting points of two pulses. ( b ) PPF, defined as the ratio of the amplitude (left) or area integral (right) of the 2nd I K versus that of the 1st responses, declines over increasing time intervals. The decay rates of PPF are fit with a single exponential function and the time constants ( n =9) are given in this and following figures. ( c , d ) Representative traces of I K recorded from outside-out patches of the nerve terminal in the absence (black traces, middle panels) or presence of α-dendrotoxin (DTX, blue traces, c ) or tetraethylammonium (TEA, magenta traces, d ) in response to the paired-pulse paradigms (top panels: amplitude: −80 to +30 mV; half-width: 0.3 ms in c , 0.45 ms in d ). ( e , f ) Summaries of the extent of PPF (quantified by area integral of I K ) with or without DTX ( n =6) or TEA ( n =7) over inter-pulse intervals. Error bars indicate ±s.e.m. 1st, first; 2nd, second. Full size image Given the intriguing feature of I K evoked by closely spaced APs, we reasoned that Kv facilitation (KvF) might be important for neurons to project their outputs onto the target cells. Therefore, we subsequently focused on the calyx of Held synapse, which is an axosomatic synapse capable of faithfully transmitting at ultra-fast speed (up to 1 kHz) to reliably convey interaural timing and intensity cues for sound localization in the auditory brainstem [17] , [18] , [19] , [20] . Unlike tiny presynaptic en passant boutons from the axons of other fast-spiking neurons, the large calyceal terminals are readily accessible with patch-clamp electrodes and can serve as an ideal model to study the mechanisms for KvF and its impact on presynaptic spikes and downstream synaptic signalling. Previous work has demonstrated that there are two major subtypes of Kvs at the calyces, namely low-threshold α-dendrotoxin (DTX)-sensitive Kv1s (K-LT) and high-threshold tetraethylammonium (TEA)-sensitive Kv3s (K-HT) that activate at −40 and −20 mV, and regulate the spike amplitude and width, respectively [18] , [19] , [21] , [22] , [23] . To directly test whether the two subtypes of Kvs with distinct kinetics and voltage dependence contribute to the facilitation differently, we performed paired-pulse experiments in the presence of either DTX or TEA to isolate currents mediated by K-HT ( I K-HT ) or K-LT ( I K-LT ) in the outside-out patch configuration. This recording mode eliminates potential contamination from other K + channels in distal axons and space-clamp errors associated with whole-cell recordings from morphologically complex calyces. We found both I K-HT and I K-LT exhibited prominent PPF but the profile of their PPF was clearly distinct ( Fig. 1c,d ). The PPF for I K-HT (179.6±10.2% at 1 ms) was much less than that for I K-LT (302.8±32.9% at 1 ms) and declined markedly faster ( τ =0.3 ms for I K-HT versus τ =0.6 ms for I K-LT ; Fig. 1e,f ). These results demonstrate that activity-dependent facilitation is present among many subtypes of Kvs, and differences in the characteristics of their PPF are likely because of heterogeneous gating kinetics of each subtype of Kvs. Interestingly, when brief voltage steps were introduced to the outside-out patches in between a pair of pseudo-APs at the interval of 1.2 ms where facilitation of I K was robust at −80 mV (168.8±4.4%), we found that PPF was attenuated by hyperpolarizing steps and eliminated (PPF=107.4±3.3%) at the non-physiologically low potential of −140 mV. Conversely, a small sub-threshold depolarization (10 mV) further enhanced facilitation of I K to 185.6±15.2% at −70 mV ( Fig. 2a ), indicating a priming effect of small depolarization on the magnitude of PPF. When the amplitude of pseudo-APs was increased from 100 to 150 mV while the rise and decay time remained unchanged, we found that the I K increased accordingly, however, the extent of PPF linearly decreased ( Fig. 2b,c ). Collectively, our experiments suggest that KvF is highly voltage dependent and inversely correlates with the inter-spike interval and spike amplitude, implying that previously activated Kvs may have a strong impact on the behaviour of Kvs in response to subsequent stimuli. 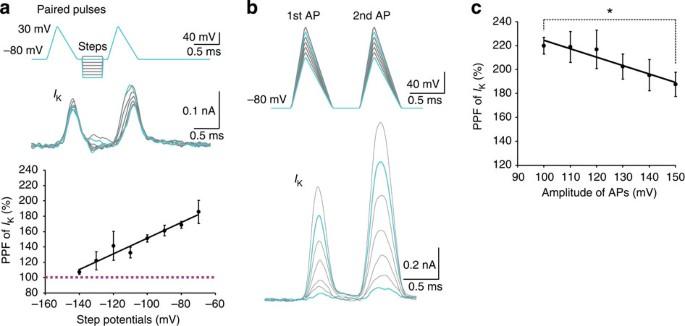Figure 2: PPF of IKdepends on the voltage and amplitude of AP-like pulses. (a)IK(middle panel) from outside-out patches triggered by paired pulses that are separated by a brief voltage step (0.4 ms) ranging from −140 to −70 mV (top panel). Note that the hyperpolarization step of −140 mV eliminates facilitation ofIKin contrast to the step of −80 mV (turquoise). Average PPF at different potentials is summarized in the bottom panel (n=5). (b) Paired pulses (top) with increasing amplitude from 100 to 150 mV used to evokeIK(bottom) from outside-out patches.IKproduced by lower (100 mV) or higher (150 mV) paired pulses are compared (turquoise). (c) The decline of PPF over the pulse amplitude is fitted with a linear regression (n=6). The asterisk indicates statistical significance (P=0.009, two-tailed paired Student’st-tests) between PPF evoked by the lower and that by the higher pulses. Error bars denote ±s.e.m. Figure 2: PPF of I K depends on the voltage and amplitude of AP-like pulses. ( a ) I K (middle panel) from outside-out patches triggered by paired pulses that are separated by a brief voltage step (0.4 ms) ranging from −140 to −70 mV (top panel). Note that the hyperpolarization step of −140 mV eliminates facilitation of I K in contrast to the step of −80 mV (turquoise). Average PPF at different potentials is summarized in the bottom panel ( n =5). ( b ) Paired pulses (top) with increasing amplitude from 100 to 150 mV used to evoke I K (bottom) from outside-out patches. I K produced by lower (100 mV) or higher (150 mV) paired pulses are compared (turquoise). ( c ) The decline of PPF over the pulse amplitude is fitted with a linear regression ( n =6). The asterisk indicates statistical significance ( P =0.009, two-tailed paired Student’s t -tests) between PPF evoked by the lower and that by the higher pulses. Error bars denote ±s.e.m. Full size image KvF is frequency dependent but Ca 2+ independent To examine whether KvF occurs during physiological activity, we recorded I K from the mature calyceal terminals using previously obtained native AP trains at various frequencies (200–400 Hz) as voltage-clamp templates ( Fig. 3 and Supplementary Fig. 3 ). Typically, these spikes displayed a slight use-dependent reduction in amplitude and persistent plateau potential resulting from depolarizing after potential (DAP) driven by resurgent Na + currents ( I Na ) [24] . 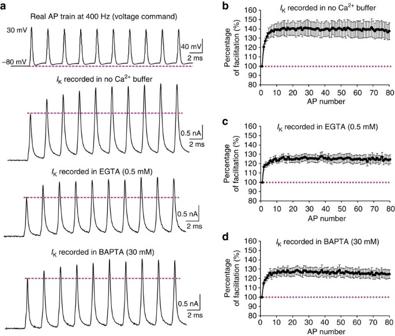Figure 3: Activity-dependent facilitation of IKis Ca2+independent. (a) Whole-cell recordings ofIKevoked by a typical presynaptic AP trains (previously obtained from the calyx of Held nerve terminal, the 1st AP has an amplitude of 110 mV, half-width of 0.28 ms and depolarizing after potential (DAP) of 9.6 mV) at 400 Hz with a duration of 200 ms (only the 1st 10 APs are shown) in the absence or presence of Ca2+buffer EGTA at low concentration (0.5 mM) or BAPTA at high concentration (30 mM). (b–d) The normalized amplitude ofIK(to the 1st response in a train) is summarized for no-Ca2+buffer (n=4,b), EGTA (n=6,c) and BAPTA (n=5,d) groups. Error bars indicate ±s.e.m. 1st, first. Figure 3a showed an example of presynaptic I K (with P/4 digital subtraction of leak and capacitive currents) evoked by 400 Hz AP trains, where the I K amplitude increased significantly in the first 5–10 spikes and sustained throughout the entire train at a level of 20–30% above the first response (first I K : 1.35±0.21 nA, 10th I K : 1.65±0.25 nA; Fig. 3c ). Such facilitation was readily reversed upon cessation of stimulation, and the magnitude of facilitation depended on the AP frequency and DAP ( Supplementary Fig. 3 ). The profile of I K facilitation was very similar to that estimated by pharmacologically isolated (that is, TEA and DTX sensitive) currents without P/N leak subtraction, indicating that this feature of Kvs cannot be attributed to the voltage-clamp errors ( Supplementary Fig. 4 ). Similar characteristics of I K were observed from hippocampal DGIs, cerebellar SNs and PCs at 22 or 35 °C ( Supplementary Fig. 1d–f ). A prominent example was SNs where realistic AP trains at 400 Hz generated >300% facilitation of I K at physiological temperature either from the whole cells or outside-out patches. In contrast, I K evoked by native APs at 50 Hz in slow-spiking CA1 neurons markedly decreased, likely as a result of use-dependent inactivation of the Kvs ( Supplementary Fig. 2 ). These results demonstrate that KvF during natural bursts of activity is frequency dependent, being most noticeable in fast neurons at high-frequency firing but largely absent in slow-spiking neurons. Figure 3: Activity-dependent facilitation of I K is Ca 2+ independent. ( a ) Whole-cell recordings of I K evoked by a typical presynaptic AP trains (previously obtained from the calyx of Held nerve terminal, the 1st AP has an amplitude of 110 mV, half-width of 0.28 ms and depolarizing after potential (DAP) of 9.6 mV) at 400 Hz with a duration of 200 ms (only the 1st 10 APs are shown) in the absence or presence of Ca 2+ buffer EGTA at low concentration (0.5 mM) or BAPTA at high concentration (30 mM). ( b – d ) The normalized amplitude of I K (to the 1st response in a train) is summarized for no-Ca 2+ buffer ( n =4, b ), EGTA ( n =6, c ) and BAPTA ( n =5, d ) groups. Error bars indicate ±s.e.m. 1st, first. Full size image Because APs not only activate Kvs but also voltage-gated Ca 2+ channels (VGCCs), which may allow Ca 2+ influx into the nerve terminal to either open Ca 2+ -gated K + channels (Kv(Ca)) or act as a second messenger to potentiate the activity of Kvs, we included Ca 2+ channel blocker CdCl 2 (20 μM) in the extracellular solution and fast Ca 2+ buffer BAPTA (30 mM) in the intracellular solution. Surprisingly, we found that these manipulations did not significantly affect the magnitude or time course of KvF as compared with the conditions where Ca 2+ buffers were omitted or only a low concentration of slow Ca 2+ buffer EGTA was present ( Fig. 3 ). Our results indicate that facilitation of I K is likely caused by use-dependent alterations in the intrinsic gating properties of Kvs, independent of VGCCs, Kv(Ca) or other Ca 2+ -dependent downstream signalling cascades. Gating kinetics of Kvs encodes activity-induced facilitation To explore the mechanisms underlying heterogeneity in KvF, we did paired-pulse experiments in Chinese hamster ovary (CHO) cell lines expressing recombinant homomeric Kv3.1 or heteromeric Kv1.1&1.2 channels, which constituted the major subunits of native Kvs [18] , [19] , [21] , [22] , [23] in the calyx of Held synapse. Simple spherical morphology of CHO cells also ensured accurate measurement of I K with minimal space-clamp errors. We found that the PPF in Kv1.1&1.2 currents was more robust (for example, PPF for Kv1.1&1.2: 495.5±55.8% versus for Kv3.1: 389.4±31.8% at the interval of 1 ms) and decayed much slower with increased inter-spike intervals than that in Kv3.1 currents ( τ =1.0 ms for Kv1.1&1.2 versus τ =0.4 ms for Kv3.1; Fig. 4a–c ), in line with the observations from native I K-HT and I K-LT in the nerve terminal ( Fig. 1 ). Most notably, the temporal onset of I K evoked by the second spikes was shifted towards to the early phase of the pseudo-spikes, as quantified by the time difference between the peak of APs and that of their evoked I K ( Fig. 4d ). The timing shift of the second I K declined exponentially over prolonged inter-spike intervals with the comparable time constants (Kv3.1: 0.4 ms versus Kv1.1&1.2: 2.4 ms; Fig. 4e,f ) to those of PPF measured by the area integral of I K ( Fig. 4c ). To investigate whether temperature has a role in KvF, we applied similar paired-pulse paradigms at 35 °C with briefer AP waveform and inter-spike intervals (−90 to 100 mV, half-width: 0.15/0.3 ms, intervals: 0.5–5 ms) to mimic realistic temperature-dependent acceleration. Although it was evident that raising temperature speeded up activation and deactivation kinetics of these channels, we noted that PPF of I K remained pronounced (for example, Kv1.1&1.2: PPF=256.2±28.0% at the interval of 1 ms; Supplementary Fig. 5 ). These results reinforce the notion that Kvs facilitate during repetitive activity regardless of their subtypes or experimental temperature. 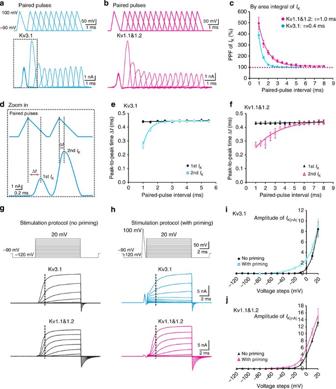Figure 4: Mechanisms underlying KvF from recombinant Kv channels. (a,b)IK(bottom panels) generated from CHO cells expressing Kv3.1 (blue,a) or Kv1.1&1.2 channels (magenta,b) by paired-pulse stimulation protocol (AP waveform: −90 to +100 mV, rise time: 0.3 ms, decay time: 0.6 ms, paired-pulse interval: 1–8 ms with increment of 0.5 ms, top panels). (c) PPF in the area integral ofIKis summarized for CHO cells transfected with Kv3.1 (blue circles,n=8) or Kv1.1&1.2 (magenta circles,n=6) constructs. The solid lines are fits to a single exponential function and time constants are shown in the figure. (d–f) The 1st pair ofIKinaare focused to show the time difference (Δt) between the peak of APs and that of correspondingIK(d). Note the marked early onset of the 2ndIKcompared to the 1stIK. Quantitative analysis of Δtare demonstrated for expression of Kv3.1 (n=8,e) or Kv1.1&1.2 (n=6,f). (g–j) Voltage steps from −120 to 20 mV (10 ms long, top panels) applied to elicitIKfrom a CHO cell expressing Kv3.1 (middle panels) or Kv1.1&1.2 (bottom panels) with (h) or without (g) the pre-pulse (−120–100 mV, rise time: 0.3 ms, decay time: 0.6 ms). The amplitude ofIKat varied potentials, measured at 2 ms after beginning of depolarization steps (dotted lines), is plotted ini(Kv3.1,n=4) andj(Kv1.1&1.2,n=4). Error bars indicate ±s.e.m. 1st, first; 2nd, second. Figure 4: Mechanisms underlying KvF from recombinant Kv channels. ( a , b ) I K (bottom panels) generated from CHO cells expressing Kv3.1 (blue, a ) or Kv1.1&1.2 channels (magenta, b ) by paired-pulse stimulation protocol (AP waveform: −90 to +100 mV, rise time: 0.3 ms, decay time: 0.6 ms, paired-pulse interval: 1–8 ms with increment of 0.5 ms, top panels). ( c ) PPF in the area integral of I K is summarized for CHO cells transfected with Kv3.1 (blue circles, n =8) or Kv1.1&1.2 (magenta circles, n =6) constructs. The solid lines are fits to a single exponential function and time constants are shown in the figure. ( d – f ) The 1st pair of I K in a are focused to show the time difference (Δ t ) between the peak of APs and that of corresponding I K ( d ). Note the marked early onset of the 2nd I K compared to the 1st I K . Quantitative analysis of Δ t are demonstrated for expression of Kv3.1 ( n =8, e ) or Kv1.1&1.2 ( n =6, f ). ( g – j ) Voltage steps from −120 to 20 mV (10 ms long, top panels) applied to elicit I K from a CHO cell expressing Kv3.1 (middle panels) or Kv1.1&1.2 (bottom panels) with ( h ) or without ( g ) the pre-pulse (−120–100 mV, rise time: 0.3 ms, decay time: 0.6 ms). The amplitude of I K at varied potentials, measured at 2 ms after beginning of depolarization steps (dotted lines), is plotted in i (Kv3.1, n =4) and j (Kv1.1&1.2, n =4). Error bars indicate ±s.e.m. 1st, first; 2nd, second. Full size image In many cases, I K evoked by the second spikes at the short intervals showed two components with clear kinks on their rise phase ( Figs 1 , 2 , 3 , 4 ). We hypothesized that activated Kvs by the first spikes may appear closed as indicated by a complete return of I K to the baseline, but actually have not recovered to the resting close state, leaving a subpopulation of Kvs in the intermediate gating states that are more willing to open. Therefore, the second spikes would result in larger I K with shorter activation latencies. To address this possibility, we used depolarization steps to measure voltage-dependent activation of Kv3.1 and Kv1.1&1.2 from CHO cells with or without a short preceding ‘priming’ spike at 22 or 35 °C ( Fig. 4g,h and Supplementary Fig. 5 ). When the amplitude of I K was plotted against the depolarizing voltages, we noticed an early onset of I K with a lower apparent activation threshold for the ‘priming’ groups, leading to a global left shift in their current ( I )–voltage ( V ) curves at both temperatures ( Fig. 4i,j and Supplementary Fig. 5 ). These observations provided direct evidence for the predictions made by previous studies [25] , [26] , which examined the effects of long-step prepulses on the gating currents of Shaker K + channels in cut-open oocytes, and implicated that intrinsic gating of K + channels might underlie the ‘Cole–Moore effect’ as first described in the squid axon [27] . We propose that this left shift in the I–V relationships by preceding AP-like activity increases the open probability of Kvs to subsequent stimuli, which gives rise to the prominent facilitation of I K in response to paired pulses or high-frequency AP bursts. Given that both native and recombinant Kvs exhibit activity-dependent facilitation, we postulated that this functional phenotype could reside in intrinsic gating kinetics of these channels. To test this, we first fit activation and deactivation kinetics of I K-HT and I K-LT recorded from the outside-out calyceal patches with the Markov modelling to derive gating rate constants [14] , [15] , [16] . We found that the classic six-state linear gating scheme (C 0 , C 1 , C 2 , C 3 , C 4 and O) fit experimental data well, and more importantly recapitulated the major characteristics of these native currents. For instance, I K-LT predicted by the model closely resembled the recorded currents in the lower activation threshold of I K following a preceding spike and paired-pulse-induced facilitation ( Fig. 5a–c ). Model fittings revealed that the backward transition rate constant ( β ) of K-LT was significantly slower than that of K-HT, whereas the forward rate constants ( α ) for both subtypes of Kvs were comparable ( Table 1 ), indicating that slower return from the intermediate closed states (C 4 …C 1 ) to resting closed state (C 0 ) may be associated with more robust facilitation of I K-LT . Indeed, when we plotted probabilities of all the kinetic states at equilibrium before the first spikes during the paired-pulse paradigm, we found that K-LT largely stayed in the C 0 and C 1 states with the other states being less dominant. The same analysis at the onset of the second pulses showed that the probability for the C 4 or O state of K-LT was very low and the C 1 state remained relatively constant at varied inter-pulse intervals. By contrast, the distribution of other closed states was highly sensitive to the intervals. As the interval was shortened (for example, <5 ms), the probability of the channel remaining in the intermediate states (C 2 and C 3 ) steeply increased at the expense of lowering the probability for the resting closed state (C 0 ). This marked re-distribution of different closed states well correlated with the time course of I K-LT facilitation ( Fig. 5c ). Taken together, we interpret our experimental and simulation results as such that the intermediate closed states of Kvs arising from previous activity decrease energy barrier to reach the open state, and hence account for accelerated activation and lowered activation threshold for Kvs susceptible to subsequent stimuli. 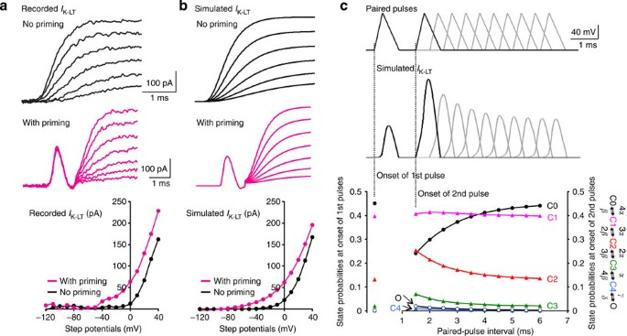Figure 5: Computer simulation of gating kinetics of Kvs. (a,b)IKrecorded from an outside-out patch of the calyx of Held nerve terminal (a) or simulated by a computational model containing five closed states and one open state (b) in response to depolarization steps from −120 to 40 mV with (magenta traces, middle panels) or without (black traces, top panels) a preceding AP-like ramp (amplitude: 110 mV; half-width: 0.45 ms). The amplitude ofIKat 2 ms after the start of voltage steps is plotted against step potentials (bottom panels) to illustrate the early activation of Kvs by the preceding depolarization. (c) Example of simulatedIK(middle) in response to a paired-pulse protocol (spike amplitude: 110 mV and half-width: 0.45 ms, paired-pulse interval: 1.5–6 ms; top). The magnitude and frequency-dependence of KvF are well reminiscent of experimental recordings ofIKas shown inFig. 1. Based on the simulation model (Table 1) with all the six states summated to 1 at any given time point during the paired-pulse paradigm, probabilities for each state of K-LT at the onset of the 1st or 2nd spikes are plotted against various inter-pulse intervals (bottom). 1st, first; 2nd, second. Figure 5: Computer simulation of gating kinetics of Kvs. ( a , b ) I K recorded from an outside-out patch of the calyx of Held nerve terminal ( a ) or simulated by a computational model containing five closed states and one open state ( b ) in response to depolarization steps from −120 to 40 mV with (magenta traces, middle panels) or without (black traces, top panels) a preceding AP-like ramp (amplitude: 110 mV; half-width: 0.45 ms). The amplitude of I K at 2 ms after the start of voltage steps is plotted against step potentials (bottom panels) to illustrate the early activation of Kvs by the preceding depolarization. ( c ) Example of simulated I K (middle) in response to a paired-pulse protocol (spike amplitude: 110 mV and half-width: 0.45 ms, paired-pulse interval: 1.5–6 ms; top). The magnitude and frequency-dependence of KvF are well reminiscent of experimental recordings of I K as shown in Fig. 1 . Based on the simulation model ( Table 1 ) with all the six states summated to 1 at any given time point during the paired-pulse paradigm, probabilities for each state of K-LT at the onset of the 1st or 2nd spikes are plotted against various inter-pulse intervals (bottom). 1st, first; 2nd, second. Full size image Table 1 Computational simulation of Kvs. Full size table KvF reduces AP amplitude and plateau potential of AP trains Lacking ideal blockers, which only inhibit activity-dependent facilitation of Kvs without affecting their basal properties, precluded us from pharmacologically examining the physiological roles of KvF in high-frequency spiking. To overcome this difficulty, we performed computer simulations by creating a modified Hodgkin–Huxley (H–H) [1] model cell (capacitance 6 pF and resting potential −80 mV) containing four components (that is, potassium conductance ( g K-HT and g K-LT ), leak conductance ( g L ) and sodium conductance ( g Na ; Fig. 6a,b ), where g K-HT , g K-LT , g L and g Na were free variables and APs were initiated by a brief inward square current (2 nA) [16] , [28] . The gating kinetics of g Na was established by fitting activation, deactivation and inactivation of I Na obtained from the outside-out patches near the heminode region of calyceal terminals ( Supplementary Fig. 6 ). Subsequently, we incorporated this conductance along with two components of Kvs derived from the Markov model into the modified H–H model cell, and produced AP trains that had the similar waveform to those realistic spikes recorded from the nerve terminal and as well as frequency-dependent adaptation (200–600 Hz; Figs 6b and 7a–c ). 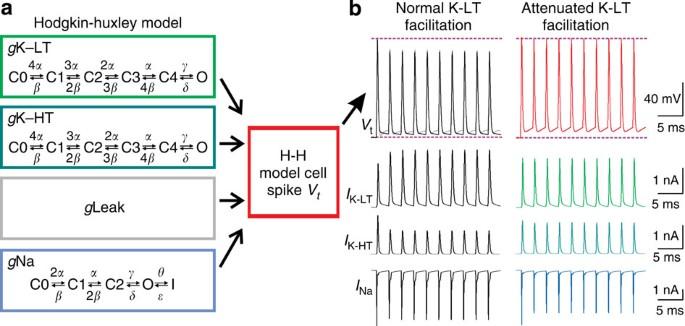Figure 6: Specific contribution of KvF to AP trains in a modified H–H model cell. (a) A modified Hodgkin–Huxley (H–H) model containing four components, that is, potassium (both low- (gK-LT) and high-threshold (gK-HT)), leak (gLeak) and sodium (gNa) conductance, wheregK-LT,gK-HT,gLeak andgNa are free variables while APs are evoked by brief current injections (2 nA, 0.2 ms). (b) Simulated AP trains at 400 Hz (top panels) before (left) and after (right) attenuating facilitation ofIK-LTby manipulating a single parametercin the rate constantβ(Table 2). The underlying currents for these two different patterns of APs are shown in the following panels. A recorded realistic AP train (grey) is included in the top left panel to illustrate its close resemblance to the simulated one. Note that attenuation ofIK-LTfacilitation increases the spike amplitude and inter-spike potential. Figure 6b showed a simulated 400 Hz train, during which I K-LT but not I K-HT facilitated greatly, consistent with the experimental evidence of their distinct decay time courses for PPF ( Fig. 1e,f ). As revealed by our model ( Fig. 5 ), fast deactivation kinetics of I K-HT might account for the lack of facilitation, particularly when evoked by a real AP train with use-dependent reduction in the amplitude. To specifically delineate the function of facilitation of I K-LT , we manually adjusted the deactivation rate constant β ( Table 2 : parameter c ) until activity-dependent facilitation was largely removed while the amplitude of the first I K-LT was maintained by increasing its total conductance. Under these conditions, we disclosed that attenuation of I K-LT facilitation eliminated activity-dependent reduction in the spike amplitude and elevated the plateau potential in the AP train ( Fig. 6b ). Surprisingly, I Na derived from the model cell with minimal I K-LT facilitation showed more prominent use-dependent inactivation, and yet remained sufficient to drive the spikes to higher amplitude. Activity-dependent decrease in the spike amplitude has classically been viewed as a result of Na + channel inactivation [2] , [7] , [11] ; however, the last line of our simulation results suggests that I K-LT facilitation can have an active role in regulating the AP amplitude by counteracting I Na during repetitive activity. Figure 6: Specific contribution of KvF to AP trains in a modified H–H model cell. ( a ) A modified Hodgkin–Huxley (H–H) model containing four components, that is, potassium (both low- ( g K-LT) and high-threshold ( g K-HT)), leak ( g Leak) and sodium ( g Na) conductance, where g K-LT, g K-HT, g Leak and g Na are free variables while APs are evoked by brief current injections (2 nA, 0.2 ms). ( b ) Simulated AP trains at 400 Hz (top panels) before (left) and after (right) attenuating facilitation of I K-LT by manipulating a single parameter c in the rate constant β ( Table 2 ). The underlying currents for these two different patterns of APs are shown in the following panels. A recorded realistic AP train (grey) is included in the top left panel to illustrate its close resemblance to the simulated one. Note that attenuation of I K-LT facilitation increases the spike amplitude and inter-spike potential. 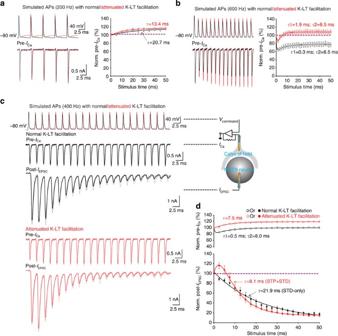Figure 7: Strong impact of KvF on synaptic input–output relationship. (a,b) Representative recordings of presynaptic Ca2+currents (pre-ICa, bottom) from the calyces elicited by simulated AP trains (top) at 200 Hz (a) or 600 Hz (b) before (black traces), and after (red traces) attenuating K-LT facilitation. The amplitude of pre-ICais normalized (Norm.) to that of the 1st pre-ICaduring the train stimuli and plotted against stimulus time (the time for the 1st AP stimulation is set as zero). The solid lines in the right panels are fits to a single or double exponential function and the time constants are given (n=9 for 200 Hz andn=6 for 600 Hz group). (c) Simultaneous recordings of pre-ICa(middle) and excitatory postsynaptic currents (post-IEPSC, bottom) from the calyx of Held synapse repeatedly evoked by simulated spikes at 400 Hz (top) with normal (grey traces) or attenuated (pink traces) K-LT facilitation. Average traces of five repeats for each group are highlighted in black or red. Recording configuration is depicted on the right. (d) The amplitude of pre-ICa(top) over 400 Hz train stimuli is fitted with a single/dual exponential function as shown with the solid lines. The post-IEPSC(bottom) are described by a single (black line, with normal K-LT facilitation) or double (red line, with attenuated K-LT facilitation) exponential function (n=8 for each group). The amplitude of both pre-ICaand post-IEPSCare normalized to that of the 1st response in a train and plotted against stimulus time. Error bars indicate ±s.e.m. 1st, first. Full size image Figure 7: Strong impact of KvF on synaptic input–output relationship. ( a , b ) Representative recordings of presynaptic Ca 2+ currents (pre- I Ca , bottom) from the calyces elicited by simulated AP trains (top) at 200 Hz ( a ) or 600 Hz ( b ) before (black traces), and after (red traces) attenuating K-LT facilitation. The amplitude of pre- I Ca is normalized (Norm.) to that of the 1st pre- I Ca during the train stimuli and plotted against stimulus time (the time for the 1st AP stimulation is set as zero). The solid lines in the right panels are fits to a single or double exponential function and the time constants are given ( n =9 for 200 Hz and n =6 for 600 Hz group). ( c ) Simultaneous recordings of pre- I Ca (middle) and excitatory postsynaptic currents (post- I EPSC , bottom) from the calyx of Held synapse repeatedly evoked by simulated spikes at 400 Hz (top) with normal (grey traces) or attenuated (pink traces) K-LT facilitation. Average traces of five repeats for each group are highlighted in black or red. Recording configuration is depicted on the right. ( d ) The amplitude of pre- I Ca (top) over 400 Hz train stimuli is fitted with a single/dual exponential function as shown with the solid lines. The post- I EPSC (bottom) are described by a single (black line, with normal K-LT facilitation) or double (red line, with attenuated K-LT facilitation) exponential function ( n =8 for each group). The amplitude of both pre- I Ca and post- I EPSC are normalized to that of the 1st response in a train and plotted against stimulus time. Error bars indicate ±s.e.m. 1st, first. Full size image Table 2 Kinetic parameters for simulating spike trains using the modified H–H model with normal or attenuated K-LT facilitation. Full size table KvF modulates short-term synaptic plasticity To elucidate functional consequences of activity-induced facilitation of Kvs, we recorded presynaptic Ca 2+ currents ( I Ca ) from the calyx of Held nerve terminal by applying the simulated presynaptic spike trains as voltage-clamp command templates with normal or attenuated I K-LT facilitation. We found that attenuation of KvF had little effect on the amplitude of I Ca by the first APs, but significantly enhanced I Ca and Ca 2+ -dependent facilitation of I Ca by subsequent APs in a frequency-dependent manner ( Fig. 7a–d ). Most strikingly, it converted depression of I Ca to potentiation at 400 or 600 Hz, demonstrating a profound impact of I K-LT facilitation on the magnitude and time course of short-term plasticity in I Ca . Given that quantal output of any given synapse is a power function of I Ca [29] , [30] , [31] , one can readily predict that the amount of transmitter release would be markedly affected. To this end, we made simultaneous paired recordings of I Ca and excitatory postsynaptic currents ( I EPSC ) from the calyx of Held synapse. When the AP template with normal I K-LT facilitation was repeatedly applied to the calyces, we found that short-term depression (STD) in I EPSC dominated at 400 Hz, consistent with previous observations from this synapse in response to afferent stimulation [32] . By contrast, when the template with attenuated I K-LT facilitation was delivered to the same nerve terminals, we noted substantial short-term potentiation (STP) of I EPSC in the early phase of the train stimulation (maximal potentiation: 115.8±6.2%), followed by a more profound and rapid STD while the first I EPSC for both sets of AP templates were not different (decay time constant of STD: 22.1±3.9 versus 7.9±0.5 ms for normal and attenuated I K-LT facilitation, respectively; Fig. 7c,d ). Unlike highly plastic synapses with heterogeneous release probability [33] , trail-to-trail fluctuations in I EPSC evoked by the same stimulation templates at the calyx of Held synapse were small ( Fig. 7c ) as a consequence of a relatively large number of release sites and size of the readily releasable pool (RRP) of synaptic vesicles (SVs) [17] . In addition to increased AP amplitude after the first spike when I K-LT facilitation was attenuated, elevated plateau potential between spikes might have also amplified the effects of higher residual Ca 2+ buildup and accelerated STD, as suggested by the previous studies showing a strong impact of small depolarization on the quantal output [34] , [35] , [36] . Taken together, our results demonstrate that these seemingly subtle changes in spike amplitude and plateau potential due to KvF converge to effectively constrain Ca 2+ influx and residual accumulation of Ca 2+ during AP bursts, leading to significant alterations in the polarity and magnitude of short-term synaptic plasticity. Given the finite number of SVs in the RRP at central synapses, we suggest that presynaptic KvF may be important for effectively conserving the RRP to sustain adequate quantal output during high-frequency neurotransmission. Presynaptic KvF promotes high-fidelity of postsynaptic spiking To directly test the physiological significance of KvF observed from the calyx of Held nerve terminal, we made dynamic-clamp recordings to examine the firing patterns of their postsynaptic neurons in response to two sets of conductance templates (STD-only versus STP+STD), derived from native I EPSC elicited at 400 Hz with normal or attenuated I K-LT facilitation ( Fig. 7c ). We first generated such digital templates by converting I EPSC into synaptic conductance (Gsyn) and then directly fed them into the postsynaptic neurons via patch electrodes. These conductances were reminiscent of realistic synaptic inputs with trial-to-trail fluctuations in the respective cases where I K-LT facilitation was present or largely absent. Notwithstanding the variability among five individual sweeps within the same groups, on average the STD-only and STP+STD templates produced distinct firing patterns ( Fig. 8a–d ). When the STD-only templates were applied, spikes were evoked reliably by the first eight stimuli before failures appeared in an alternating manner ( Fig. 8e,h ; spike failure rate: 36.7±2.4%), typical of the phase-locking phenotype of these native neurons [20] . In contrast, when stimulated with the STP+STD templates, the same neurons fired much fewer consecutive spikes early in the train and subsequently failed to generate spikes completely ( Fig. 8f,h ; spike failure rate: 52.9±1.6%). Quantitative analyses of the time difference between the peak of the seventh APs and that of the seventh current inputs showed a substantial delay in the spike latency for the STP+STD paradigm (0.95±0.06 ms) as compared with the STD-only template (0.72±0.02 ms; Fig. 8g,i ). Collectively, this evidence denotes that facilitation of presynaptic I K may serve as a built-in mechanism to support sustained postsynaptic spiking by dynamically attenuating presynaptic Ca 2+ influx and preventing rapid depletion of the RRP during AP bursts. 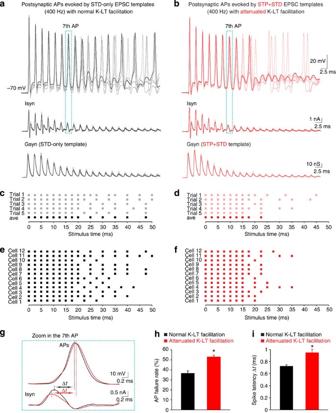Figure 8: Indispensable role of KvF in boosting spiking fidelity of principal neurons. (a,b) Conductance templates (Gsyn), STD-only (individual trials in grey and average (Ave) trial in black,a) and STP+STD (individual trials in pink and average trial in red,b) are generated by reversing the polarity of two sets of representative recordings of post-IEPSC, respectively, evoked by the train stimulation (400 Hz) with normal or attenuatedIK-LTfacilitation (bottom panels). Spikes evoked by stimulation currents (Isyn, middle panels) in the dynamic-clamp configuration by injecting the EPSC templates into the same postsynaptic neurons are shown in top panels. (c,d) APs produced by the five individual and average conductance templates for each group are summarized. Each square represents a spike. (e,f) Raster plots of APs generated by the average conductances of five repeats against stimulus time in 12 cells. (g) Time difference between the peak of the 7th stimulation currents and that of their resulting APs during the train stimuli, termed as spike latency, is illustrated to display the prolonged spike latency withoutIK-LTfacilitation. (h,i) Failure rate (h) and latency (i) of spikes produced by the STD-only (black bars) or STP+STD template (red bars) are compared (n=12). The asterisks indicate statistical significance (P<0.0001 in both cases, two-tailed paired Student'st-tests). Error bars denote ±s.e.m. Figure 8: Indispensable role of KvF in boosting spiking fidelity of principal neurons. ( a , b ) Conductance templates (Gsyn), STD-only (individual trials in grey and average (Ave) trial in black, a ) and STP+STD (individual trials in pink and average trial in red, b ) are generated by reversing the polarity of two sets of representative recordings of post- I EPSC , respectively, evoked by the train stimulation (400 Hz) with normal or attenuated I K-LT facilitation (bottom panels). Spikes evoked by stimulation currents ( I syn, middle panels) in the dynamic-clamp configuration by injecting the EPSC templates into the same postsynaptic neurons are shown in top panels. ( c , d ) APs produced by the five individual and average conductance templates for each group are summarized. Each square represents a spike. ( e , f ) Raster plots of APs generated by the average conductances of five repeats against stimulus time in 12 cells. ( g ) Time difference between the peak of the 7th stimulation currents and that of their resulting APs during the train stimuli, termed as spike latency, is illustrated to display the prolonged spike latency without I K-LT facilitation. ( h , i ) Failure rate ( h ) and latency ( i ) of spikes produced by the STD-only (black bars) or STP+STD template (red bars) are compared ( n =12). The asterisks indicate statistical significance ( P <0.0001 in both cases, two-tailed paired Student's t -tests). Error bars denote ±s.e.m. Full size image Our study has established a new form of frequency-dependent but Ca 2+ -independent facilitation of Kvs, which is widely present in neurons from hippocampus, cerebellum and auditory brainstem. Particularly relevant to the physiological functionality of fast synapses such as the calyx of Held synapse, facilitation of presynaptic I K-LT attenuates the spike amplitude and inter-spike potential during high-frequency bursts. It impacts the magnitude and polarity of short-term plasticity in presynaptic Ca 2+ inflow and transmitter release, ultimately enhancing the fidelity of postsynaptic spiking ( Figs 7 and 8 ). Given a limited size of the RRP in the nerve terminal, we suggest that frequency-dependent attenuation in spike amplitude and inter-spike potential by facilitating Kvs is an indispensable adaptation for the efficient usage of release-competent SVs to maintain sustained synaptic drive. Such a mechanism enhances the phase-locking phenotype of the calyx of Held synapse, which is critical for sound localization [20] . Extrapolating from this proof of principle at the calyx of Held synapse, we suggest that similar frequency-dependent facilitation of Kvs at the axons or boutons of other fast-spiking central neurons may restrain depletion of SVs in the RRP and help improve sustainability of neurotransmission at high-frequency neural activity. Unlike Ca 2+ -dependent facilitation of VGCCs through calmodulin binding to VGCCs or facilitation of Kv(Ca) by Ca 2+ binding to their own EF motifs [37] , [38] , we have found that facilitation of Kvs exclusively results from the intrinsic gating kinetics of these channels in transition between the intermediate closed states and the open state during repetitive activity. Similar features of Kvs from several native neurons and mammalian cell lines expressing recombinant Kv1.1&1.2 or Kv3.1 channels reinforce the view that Kvs express facilitation without other endogenous modulators, despite that low- and high-threshold Kvs bear different extent and dynamics of facilitation. In the squid axon, Cole and Moore [27] first described that hyperpolarization of membrane potential slowed down activation of I k . It initiated the debate whether this so-called ‘Cole–Moore effect’ lay in the channel gating itself or could be resulted from more than one types of K + channels with distinct activation kinetics and voltage dependence in the squid axon [39] , [40] , [41] . Subsequent studies on the voltage dependence of gating currents (that is, generated by the charge transfer of voltage sensor) in cut-open oocytes expressing homomeric Shaker channels demonstrated that the ‘Cole–Moore effect’ could be accounted for by the gating itself [25] , [26] . Using both native Kvs in nerve terminals and homogeneous recombinant Kvs in cell lines, we have provided concrete evidence that preceding depolarization can accelerate activation of Kvs as a result of a left shift in the I – V curve and lead to a facilitation of I k ( Figs 1 , 2 , 3 , 4 ). By applying the Markov modelling of Kv kinetics including six gating states ( Fig. 5 ), we have further revealed that the key determinant of the ‘Cole–Moore effect’ is the deactivation time constant ( β ) of Kvs, which likely gives rise to heterogeneity in the magnitude and time course of facilitation. We interpret our observations as such that preceding activity shifts a relative fraction of Kvs to different intermediate closed states of the same channels. Compared with the resting closed state (C 0 ), the intermediate closed states (C 1 –C 4 ) have lower energy barrier to reach the open state (O) and hence display a lower activation threshold and faster activation kinetics. Although the ‘Cole–Moore effect’ has been intensively debated as an interesting biophysical phenomenon since 1960s, its physiological relevance remains unknown. Our study brings to light the significant roles of the ‘Cole–Moore effect’, more specifically, the intermediate closed states of Kvs, in determining presynaptic AP waveform and short-term synaptic plasticity. We suggest that the classical ‘Cole–Moore effect’ of Kvs can fully account for I k facilitation in repetitive firing at the calyx of Held nerve terminal and perhaps other fast-spiking neurons [42] , [43] . Instead of standard square voltage steps, we have used AP-like ramps or real APs to explore the gating behaviours of Kvs and their activity-dependent facilitation. In a few studies, where AP waveforms had been applied to cortical neurons, Kvs appeared to undergo use-dependent inactivation during high-frequency trains, leading to frequency-dependent spike broadening [35] , [44] , [45] . Such a discrepancy may be because of the differences in the AP waveform as well as composition of Kvs associated with different neuronal populations, as we have demonstrated that KvF is strongly dependent on the AP amplitude, voltage and subtype of Kvs ( Figs 1 and 2 ). Fast-spiking neurons characterized in this study usually contain delayed rectifier Kvs such as Kv3.1 and Kv1.1/1.2 that show little inactivation. High density of these fast-gating delayed rectifiers instates brief APs and minimizes use-dependent reduction in the spike amplitude during high-frequency firing to promote the manifestation of I K facilitation. Conversely, in slow-spiking neurons, such as hippocampal CA1 neurons, rapid inactivating Kvs (for example, A-type currents or C-type inactivation) may dominate and cause severe use-dependent adaptation of spikes, during which the functional expression of KvF can be masked, albeit the fact that these channels do facilitate in response to closely adjacent APs ( Supplementary Fig. 2 ). It is worth noting that use-dependent decline in the spike amplitude during repetitive activity has traditionally been attributed to rapid inactivation of Na + channels. Surprisingly, under our simulation environment, frequency-dependent facilitation of Kvs actively contributes to the attenuation of the AP amplitude and DAP by counteracting I Na -induced depolarization ( Fig. 6 ). Hence, KvF may become another factor to be considered for interpreting complex AP firing patterns at high rates in addition to classical inactivation of Na + channels. By paired recordings from pre- and postsynaptic compartments of the calyx of Held synapse, we further demonstrate that the subtle decrease in the spike amplitude and inter-spike plateau potential because of facilitation of I K-LT strongly impacts I Ca and residual Ca 2+ buildup in the nerve terminal and ultimately quantal output during high-frequency train stimulation ( Fig. 7 ). It is also possible that heterogeneous levels of K-LT in morphologically distinct calyces can modulate presynaptic APs differently, leading to divergent forms of short-term facilitation and depression phenotypes as previously described [46] . Taking together, this study adds a new variable to the mechanistic underpinnings of short-term synaptic plasticity, aside from several other proposed mechanisms [17] , [47] . In summary, our experimental evidence and computer simulations have led us to conclude that neural activities prime presynaptic Kvs into the intermediate closed states before subsequent stimuli arrive, likely owing to different positions of four voltage sensors (S4) within each Kvs [13] , [48] . These sensors not only gate Kvs but also serve as direct decoders for the frequency of afferent axonal activity, which drive facilitation of I K to dampen depolarization and consequentially influence Ca 2+ -dependent short-term plasticity and postsynaptic spiking fidelity. The multifaceted function of voltage sensors may be applicable to other voltage-gated ion channels as well. Such an intrinsic mechanism of Kvs is of essential importance for fine-tuning spike waveform, inter-spike potential and synaptic input–output relationship during high-frequency neurotransmission at the calyx of Held and other fast central synapses. Slice preparation Mice were housed in the facility certified by the Canadian Council of Animal Care and were used for this study according to a protocol approved by the Hospital for Sick Children Animal Care Committee. Brainstem slices were prepared from postnatal (P) 16 to 19-day–old animals, as previously described [49] . After decapitation with a small guillotine, brains were immediately immersed into semi-frozen artificial cerebral spinal fluid (ACSF) containing (in mM): NaCl (125), KCl (2.5), glucose (10), NaH 2 PO 4 (1.25), Na-pyruvate (2), myo-inositol (3), ascorbic acid (0.5), NaHCO 3 (26), MgCl 2 (1) and CaCl 2 (2) at a pH of 7.3 when oxygenated (95% O 2 and 5% CO 2 ) followed by rapid dissection. Hippocampal and cerebella slices were taken from 6 to 8-week-old mice in ice-cold solution including (in mM): NaCl (81.2), NaHCO 3 (23.4), sucrose (69.9), glucose (23.3), KCl (2.4), NaH 2 PO 4 (1.4), MgCl 2 (6.7) and CaCl 2 (0.5) at a pH of 7.3. Transverse slices of the auditory brainstem containing the medial nucleus of the trapezoid body or parasagittal slices including cerebellum and hippocampus were cut at a thickness of 200–250 μm using a microtome (VT1000S, Leica) and incubated in ACSF at 37 °C for one hour before experimentation. CHO cells expressing Kv1.1&1.2 or Kv3.1 channels CHO cells (ATCC CCL-61) were maintained in 60 mm tissue culture dishes (Nunc, Thermo Fisher Scientific) containing 5 ml of Ham’s F12 media (Wisent) supplemented with 10% fetal bovine serum and 1% penicillin-streptomycin (Wisent); and grown at 37 °C and 5% CO 2 . Cells were split twice weekly to prevent overgrowth. Cells were split by removing the culture medium, washing the cells once with 10 ml phosphate-buffered saline (Wisent) and then incubating with 1 ml trypsin–EDTA (0.25%) for 3 min at room temperature. Subsequently, 5 ml of culture medium was added to the dish, and cells were dissociated mechanically. Then 0.5 ml of medium containing dissociated cells ( ~ 2 × 10 5 cells) was added to a new dish. CHO cells (1 × 10 4 cells per cm 2 ) were plated 1 day before transfection onto coverslips coated with poly-d-lysine (50 μg ml −1 , Sigma). Transfection was carried out using the FuGene HD (Roche) method with Kv1.1-RFP:Kv1.2-GFP ratio of 1:1 (gift from Drs Gang Xie and John Roder, University of Toronto). After transfection, cells were maintained in Ham’s F12 media for 48 h before experiments. CHO cells with stable expression of Kv3.1 channels were generously provided by Dr Leonard K Kaczmarek (Yale University). Electrophysiology For recordings from brain slices, ACSF was supplemented with bicuculline (10 μM) and strychnine (1 μM) to block inhibitory inputs. To isolate K + currents, TTX (0.5 μM) and CdCl 2 (20 μM) were added to block Na + and Ca 2+ channels. Intracellular solution for recording K + currents and APs contained the following (in mM): K-gluconate (97.5), KCl (32.5), EGTA (0.5) or BAPTA (30), HEPES (40) and MgCl 2 (1), pH 7.3. To isolate presynaptic Ca 2+ currents, TTX (0.5 μM), TEA (10 mM), and 4-aminopyridine (0.3 mM) were applied extracellularly to inhibit Na + and K + channels. Intracellular solution for recording presynaptic Ca 2+ currents included (in mM): CsCl (110), HEPES (40), EGTA (0.5), MgCl 2 (1), ATP (2), GTP (0.5), phosphocreatine (12), TEA (20) and K-glutamate (3), pH adjusted to 7.3 with CsOH. For postsynaptic recordings, intracellular solution contained (in mM): K-gluconate (97.5), CsCl (32.5), EGTA (5), HEPES (10), MgCl 2 (1), TEA (30) and lidocaine N -ethyl bromide (3), pH 7.3. Patch electrodes typically had resistances of 4–6 and 2.5–3 MΩ for pre- and postsynaptic recordings, respectively. For whole-cell voltage-clamp recordings, pre- and postsynaptic series resistances were 6–15 MΩ (<10 MΩ in most cases) and 3–6 MΩ, respectively, and compensated to 90%. The respective holding potential for pre- or postsynaptic neurons was −80 and −60 mV. Presynaptic K + and Ca 2+ currents were evoked by the voltage-command protocols indicated in the text, and leak subtraction was done with an online P/4 procedure. To validate the online leak P/N subtraction, we recorded raw currents evoked by a typical AP train at 400 Hz without P/N subtraction after blocking Na + channels with TTX and Ca 2+ channels with CdCl 2 . We subtracted these currents with those obtained with additional blockers for K-HT (TEA) and K-LT (DTX). By comparing the subtracted TEA and DTX-sensitive currents with K + currents recorded with online P/N correction, we found that they were almost identical in the amplitude and more importantly in the profile of facilitation over the train stimuli ( Supplementary Fig. 4 ). For experiments where real APs were used as voltage command ( Fig. 3 and Supplementary Figs 3 and 4 ), we first recorded APs from a P17 calyx at a sampling rate of 50 kHz in current-clamp configuration by stimulating afferent axon fibres using a bipolar platinum electrode delivered through a stimulator (Master-8, A.M.P. Instruments). After manually removing stimulation artefacts preceding the APs, the digitized values were fed back into the amplifier as voltage-command templates (Axon Text File) through pClamp 9 software (Molecular Devices) at the same sampling frequency as their acquisition. Similarly, the current-command templates in Fig. 8 were generated by reversing the polarity of previously obtained EPSCs in response to 400 Hz train stimuli with normal or attenuated K-LT facilitation ( Fig. 7 ) and converting these currents to conductance by G = I /( V m − E rev ), where V m and E rev were set at −70 and 0 mV, respectively, for postsynaptic neurons. The digitized conductance templates (Text File) were injected into these neurons to evoke APs with an amplifier (AXOPATCH 200B, Molecular Devices) and a digitizer (CED 1401, Cambridge Electronic Design). CHO cells transfected with Kv1.1&1.2 were positively identified with red/green fluorescence illuminated briefly by a mercury burner (Olympus). Recordings from CHO cells expressing Kv3.1 or Kv1.1&1.2 ( Fig. 4 and Supplementary Fig. 5 ) were made in the extracellular solution containing (in mM): NaCl (140), KCl (2.5), CaCl 2 (1.3), HEPES (10) and glucose (33), pH 7.3. And the intracellular solution was the same as used for recording K + currents from brain slices. The holding potential was set at −90 mV and series resistance was 3–6 MΩ, compensated to 90%. Most of the electrophysiological experiments were performed at room temperature (~22 °C), except for several sets of recordings of K + currents from CHO cells or cerebellar neurons obtained at 35 °C using an inline heater with a feedback thermistor (TC-324B, Warner Instruments). All the recordings (except for those in Fig. 8 ) were acquired online, filtered at 4 kHz, digitized at 50 or 100 kHz with a dual-channel amplifier (MultiClamp 700A, Molecular Devices) and digitizer (Digidata 1322A, Molecular Devices). Reagents were obtained from Sigma (St Louis, MO), Tocris Cookson (Bristol, UK) and Alomone Labs (Jerusalem, Israel). Data analysis Data were analysed offline with pClamp 9 (Molecular Devices), MiniAnalysis (Synaptosoft) and Excel XP (Microsoft). PPF was calculated by dividing the amplitude or area integral of the second K + current by that of the first one during a paired-pulse stimulation. The decay time course of PPF over increasing paired-pulse intervals was described with a single exponential function: f( t )=∑ A *exp(− t / τ )+ C . Time constants ( τ ) were given in respective figures. In Fig. 7 , the amplitude of I Ca and I EPSC elicited by each AP train was normalized to that of the first currents. The time course of normalized I Ca and I EPSC over an AP train was fitted with a single or double exponential function. Statistical tests of significance were two-tailed, paired Student's t -tests with a P value cutoff of <0.05. Data were expressed as the mean±s.e.m from a population of cells ( n ). Computer simulations Kinetic fittings of activation and deactivation of I K-HT , I K-LT and I Na from outside-out patches in voltage-clamp experiments were performed using the Markov model in combination with particle swarm optimization and golden section search-based algorithms to determine the optimal match to macroscopic currents and to extract all free-rate parameters ( Table 1 and Supplementary Fig. 6 ). Details of computational methods were previously described [16] , [28] . All conductances were incorporated into the modified H–H model cell for simulating APs at different frequencies. The differential equations for the kinetic modelling were solved numerically, using a fifth-order Runge–Kutta integration method. The integrating routines were written and executed with software CeL (Huazhong University of Science and Technology, Wuhan, China) and compiled with the C++ compiler to run under Windows XP ( www.HustCeL.com ). How to cite this article: Yang, Y.-M. et al . Enhancing the fidelity of neurotransmission by activity-dependent facilitation of presynaptic potassium currents. Nat. Commun. 5:4564 doi: 10.1038/ncomms5564 (2014).